Motor deficits seen in microglial ablation mice could be due to non-specific damage from high dose diphtheria toxin treatment 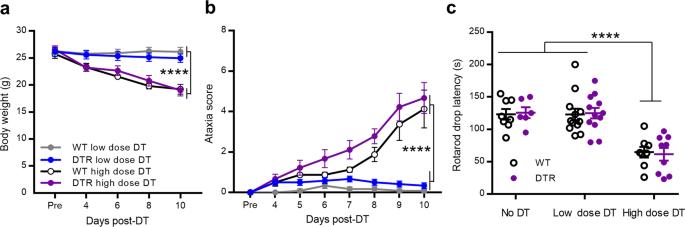Fig. 1: High dose diphtheria toxin non-specifically induced motor deficits. aBoth WT (n= 8) and CX3CR1CreER/+/R26iDTR/+(DTR) (n= 9) mice showed similar and significant body weight decrease after high dose DT (1.0 μg × 3) treatment. While both groups of low dose DT (0.5 μg×2) (n= 12 for each group) treated mice maintained stable body weight within two weeks. (two-way ANOVA with repeated measurement,F(3, 37) = 7.763, ***p= 0.0004 for group effects.p= 0.5985 between WT and DTR high dose groups,p= 0.5465 between WT and DTR low dose groups.).bAtaxia score assessment showed significant progressive ataxia behavior in both WT and DTR mice with high dose DT treatment; In the low dose DT treated groups, 5/12 WT and 10/12 DTR mice transiently showed slight ledge walking problem (score 1), and most of the mice fully recovered in the last observation (score 0, 4/5 WT, and 8/10 DTR mice); other low dose DT-treated mice remained normal (score 0) all the time. Mouse numbers were equal to panelafor each group (two-way ANOVA with repeated measurement,F(3, 37) = 22.74, ****p< 0.0001, for overall group effects.p= 0.2425 between WT and DTR high dose groups,p= 0.0025 between WT and DTR low dose groups andp> 0.3 for day 8 and later with post-hoc Sidak’s test, two sides.).cRotarod test showed significant shorter drop latency for both high dose DT-treated WT and DTR mice comparing to no DT-treated controls (n= 8 for WT control,n= 6 for DTR control). While both low dose DT-treated groups showed similar rotarod performance as controls (****p< 0.0001, un-pairedt-test, two sides). All the DT-treated mouse were used for data collection of (a–c). Data were presented as mean ± SEM. Source data are provided as a Source Data file for (a–c). 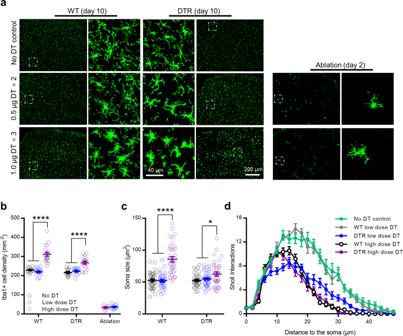Fig. 2: High dose diphtheria toxin non-specifically induced microglia activation. aRepresentative Iba1 staining images from cortex. The enlarged images were from the areas indicated by the square frame of each group.bCortical Iba1+ microglial cell densities showed that low dose DT (n= 16) treatment did not alter microglia density in the WT mice, but high dose (n= 19) significantly increased the density compared with no DT WT control (n= 12); Repopulated microglia in the low dose DT (n= 14) treated DTR mice reached basal cell density (n= 12) at 10 days, but was significantly increased in the high dose DT (n= 18) group. The microglia depletion efficiencies between the high (n= 8) and lose dose (n= 10) DT groups were comparable. (****p< 0.0001,t-test, two sides).cSoma size measurement showed dramatic cell body enlargement in the high dose (n = 36) but not low dose DT (n= 36) treated WT mice, and in the high dose (n= 36) but not low dose DT (n= 36) treated DTR mice (n= 36 for no DT WT,n= 33 for no DT DTR group, ****p< 0.0001, *p= 0.0129,t-test, two sides).dSholl analysis of individual Iba1+ microglia cells showed that the low dose DT (n= 13) treatment in WT mice did not alter microglia morphology compared with no DT controls (n= 17, WT and DTR control data were pooled together,p= 0.9837). Microglia from both high dose DT treated WT (n= 17) and DTR (n= 16) mice showed similar less interactions than no DT controls (p< 0.0001). Microglia from the low dose DT treated DTR (n= 14) mice also showed less interactions than no DT controls (p< 0.0001) Two-way ANOVA with repeated measurement (b–d, images collected from 3 mice for each group, exceptn= 5 mice for the low dose DT ablation at 2 days). Data were presented as mean ± SEM. Source data are provided as a Source Data file for (b–d). Animals All experimental procedures were approved by the Institutional Animal Care and Use Committee of Nanchang University. We followed the guidelines set forth by the Guide of the Care and Use of Laboratory Animals 8th Edition. CX3CR1-CreER (#021160) mice and ROSA26-iDTR (#007900) mice were origin from the Jackson laboratory. Wild type C57BL6/N mice were obtained from SLAC Laboratory Animal Co. Ltd. Only male mice were used for the whole study. The genotypes were blinded to the experimenters. Mice were group (4–5 per cage) housed in 12/12 light/dark cycle, 23 ± 1 °C vivarium environment. Food and water were available ad libitum . Tamoxifen (150 mg/kg, 20 mg/ml in corn oil, 4 i.p. injections with 48 h intervals; Sigma) was injected into 6–8 weeks old CX3CR1 CreER/+ /R26 iDTR/+ mice to induce DT receptor expression in microglia. DT injection was done at 3 weeks after the last tamoxifen treatment. DT administration New DT (Merck Millipore, #322326) was prepared as a 100 μg/ml stock solution in PBS, separated into tubes of 100 μl volume and stored at −20 °C. The stock solution was diluted to 5 μg/ml for the high dose injection and 2.5 μg/ml for the low dose injection. All DT injections were done within 2 weeks after the stock preparation. Fresh diluted solution was used immediately, and the remaining was discarded. Behavioral assessment Ataxia scoring was assessed according to a previous published protocol that was used by the criticized paper as well [14] . Ledge test monitored the mice walking along the cage ledge; Hindlimb clasping monitored the hindlimb posture when the mice were held by the tail. Gait assessed the hindlimb walking performance. Kyphosis assessed the dorsal curvature of the spine. Each individual test was scored on a scale of 0–3 with 0 representing normal and 3 being the most severe manifestation. All 4 scores were added together as the final score. Each test was performed at least 3 times. Rotarod tests were performed on an accelerated Rotarod (30 mm in diameter, www.softmaze.com ). The mice were first placed on the rotarod with 5 RPM speed for 5 min habituation. For the test, the speed started from 0 RPM, and accelerated to 60 RPM in 300 s. The time latency that mice fell from the rotarod was recorded. Fluorescent immunostaining Mice were deeply anaesthetized with isoflurane (5% in O 2 ) and perfused transcardially with 20 ml PBS followed by 20 ml of cold 4% paraformaldehyde (PFA) in PBS. The whole brain was removed and post-fixed with the same 4% PFA for 4–6 h at 4 °C. The samples were then transferred to 30% sucrose in PBS for at least 48 h in dark conditions. Sample sections (18 μm in thickness) were prepared on gelatin-coated glass slide with a cryostat (Leica). The sections were blocked with 5% goat serum and 0.3% Triton X-100 (Sigma) in TBS buffer for 45 min, and then incubated overnight at 4 °C with a primary antibody for rabbit-anti-Iba1 (1:800, Abcam, Catalog ab178846). The sections were then incubated for 90 min at room temperature, with secondary antibodies (1:500, Alexa Fluor 546, Life Technologies, Catalog A-21085). The sections were mounted with Fluoroshield™ with DAPI (Sigma). Fluorescent images were obtained with a confocal microscope (Olympus). Cell counting, soma size and sholl analysis were quantified using the ImageJ software (ImageJ 1.52a, National Institutes of Health, Bethesda, MD). Statistical analysis Data were presented as mean ± SEM. Student’s t -test and ANOVA test were performed using GraphPad (GraphPad Prism 7, GraphPad software Inc.) to establish significance. * p < 0.05, **p < 0.01, *** p < 0.001. Reporting summary Further information on research design is available in the Nature Research Reporting Summary linked to this article.